Rare coding variants and X-linked loci associated with age at menarche More than 100 loci have been identified for age at menarche by genome-wide association studies; however, collectively these explain only ∼ 3% of the trait variance. Here we test two overlooked sources of variation in 192,974 European ancestry women: low-frequency protein-coding variants and X-chromosome variants. Five missense/nonsense variants (in ALMS1 / LAMB2 / TNRC6A/TACR3/PRKAG1 ) are associated with age at menarche (minor allele frequencies 0.08–4.6%; effect sizes 0.08–1.25 years per allele; P <5 × 10 −8 ). In addition, we identify common X-chromosome loci at IGSF1 (rs762080, P =9.4 × 10 −13 ) and FAAH2 (rs5914101, P =4.9 × 10 −10 ). Highlighted genes implicate cellular energy homeostasis, post-transcriptional gene silencing and fatty-acid amide signalling. A frequently reported mutation in TACR3 for idiopathic hypogonatrophic hypogonadism (p.W275X) is associated with 1.25-year-later menarche ( P =2.8 × 10 −11 ), illustrating the utility of population studies to estimate the penetrance of reportedly pathogenic mutations. Collectively, these novel variants explain ∼ 0.5% variance, indicating that these overlooked sources of variation do not substantially explain the ‘missing heritability’ of this complex trait. Age at menarche, the onset of first menstruation in females, indicates the start of reproductive maturity and is a commonly reported marker of pubertal timing. One hundred and six genomic loci for this highly heritable trait have been mapped by genome-wide association studies (GWAS), implicating many previously unsuspected mechanisms [1] . However, to date that approach has been limited to consideration of only those genetic variants captured by autosomal HapMap2 reference panels. In particular, like most GWAS for other complex traits, previous GWAS for age at menarche provided poor coverage for low-frequency variants and omitted sex chromosome data. Here we report a dual strategy for assessing genetic variation overlooked by those prior efforts: low-frequency protein-coding variants genotyped by large-scale exome-focussed arrays and high-density X-chromosome single-nucleotide polymorphism (SNP) genotyping and imputation. We identify several new associations between rare protein-coding and X-linked variants with age at menarche in women of European ancestry. The findings implicate new mechanisms that regulate puberty timing, but collectively these novel variants explained only ∼ 0.5% of the variance, indicating that these often overlooked sources of variation that do not substantially explain the ‘missing heritability’ of this complex trait. 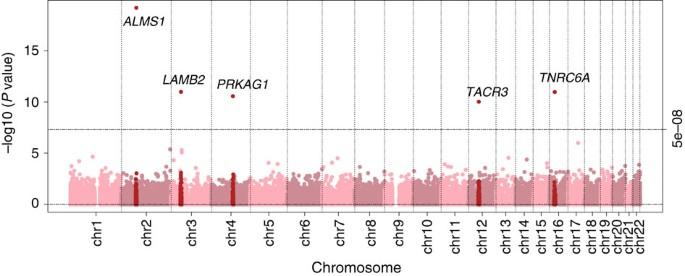Figure 1: A ‘Manhattan plot’ of menarche association statistics for the genotyped low-frequency exome array variants. Test statistics are shown from the exome-chip discovery-phase samples, with the exception of the five labelled loci that indicate results from the combined discovery and replication set. From the exome array studies, 61,734 low-frequency (minor allele frequency (MAF) <5%) variants passed quality-control (QC) criteria in a combined sample of up to 76,657 women of European ancestry from 19 studies ( Supplementary Table 1 ). Gene-based burden and SKAT tests that aggregate the effects of variants with MAF<1% yielded no significant associations with age at menarche. A linear regression test was used to derive all P values obtained in this study. Meta-analysis of individual variant associations with questionnaire-reported variation in age at menarche (restricted to the ages of 9–17 years) in this discovery phase identified one signal at genome-wide statistical significance ( P <5 × 10 −8 ); this was a rare missense variant in the Alström’s syndrome gene ( ALMS1 , rs45501594, p.T3544S, MAF 1%; P =4.6 × 10 −10 ). For follow-up testing in up to 116,317 independent women of European ancestry from the deCODE (Diabetes Epidemiology: Collaborative analysis of Diagnostic criteria in Europe) and 23andMe studies, we selected rs45501594 and 23 other variants that met the following criteria: protein coding, present in over half of the exome array studies, and with association P <5 × 10 −4 . In the follow-up samples, 7 of the 20 variants that passed QC showed directionally concordant confirmatory associations with P <0.05, of which five reached genome-wide significance in a combined meta-analysis of discovery phase and follow-up data ( Table 1 , Fig. 1 , Supplementary Fig. 1 ). No significant heterogeneity between studies was observed at any of these loci ( Supplementary Fig. 2 ). Table 1 Association statistics for the novel low-frequency and X-chromosome variants. Full size table Figure 1: A ‘Manhattan plot’ of menarche association statistics for the genotyped low-frequency exome array variants. Test statistics are shown from the exome-chip discovery-phase samples, with the exception of the five labelled loci that indicate results from the combined discovery and replication set. Full size image The rare missense variant in ALMS1 (rs45501594, Supplementary Fig. 3 ) remained the strongest signal identified using exome array studies (combined: P =6.8 × 10 −20 ). In the follow-up samples, each rare allele was associated with 0.23-year-later age at menarche, an effect size more than double that of any genetic variant previously reported for puberty timing in the general population. This strong signal was not detected by the previous HapMap2-based GWAS as it is poorly tagged by common SNPs in that reference panel (maximum proxy SNP, r 2 =0.24). Deleterious mutations in this gene cause Alström’s syndrome (OMIM no. 203800), a rare, autosomal-recessive disorder characterized by cone–rod dystrophy, sensorineural hearing loss, dilated cardiomyopathy, childhood obesity, insulin resistance, diabetes mellitus, hypogonadotropic hypogonadism in males, menstrual irregularities and early puberty in females, and short stature in adulthood [2] . Hypogonadism was also invariably observed in an ALMS1 gene-trapped mouse model [3] . The variant with largest effect was a rare stop-gain mutation in the tachykinin receptor 3 gene ( TACR3 ; rs144292455, MAF=0.08%, combined P =2.8 × 10 −11 , Supplementary Fig. 3 ); in follow-up samples each rare allele was associated with 1.25-year-later age at menarche. Common HapMap2 SNPs at the TACR3 locus were previously associated with age at menarche [1] ; however, the rare variant rs144292455 is not tagged by the HapMap2 or conventional 1000G imputation (it was directly genotyped in 23andMe and was imputed in deCODE). Statistical independence was confirmed by observing significant association with the common TACR3 SNP in a sensitivity analysis within a participating study (Women's Genome Health Study (WGHS), Supplementary Table 1 ) that excluded rare allele carriers. The rare allele causes a premature stop codon (p.W275X) in the fifth transmembrane segment of the 465 amino-acid receptor for the neuropeptide neurokinin B, and is the most frequently reported TACR3 mutation in the rare reproductive disorder idiopathic hypogonadotropic hypogonadism (idiopathic hypogonadotropic hypogonadism (IHH), OMIM no. 614840) [4] . Both homozygous and heterozygous p.W275X variants have been reported in male IHH cases with features of ‘early androgen deficiency’; however, notably the heterozygous cases showed evidence of spontaneous neuroendocrine recovery. Our findings suggest that heterozygous p.W275X variants contribute to the normal variation in puberty timing, whereas homozygous inheritance or possibly compound heterozygosity is required for IHH. A low-frequency missense variant in the LAMB2 gene was associated with 0.08-year-later age at menarche (rs35713889, p.G914R, MAF 4%; P =1.1 × 10 −11 ; Supplementary Fig. 3 ). In the same region (3p21.31) we previously reported a HapMap2 GWAS locus for age at menarche (locus 19a and 19b in ref. 1 ); however, the low-frequency variant rs35713889 is poorly tagged by common HapMap2 SNPs (the best proxy rs1134043, r 2 =0.24, was reportedly not associated with age at menarche: P =0.35 (ref. 1 )). The strongest reported [1] HapMap2 signal at this locus is only weakly correlated with rs35713889 (rs3870341, MAF=26%; r 2 =0.07, distance 422 kb), and both signals remained significant when jointly tested in a follow-up sample of 76,831 women from the 23andMe study (in separate models: rs35713889: β =0.08 years per allele, P =0.0001 and rs3870341: β =0.04, P =4.5 × 10 −5 ; in the joint model: rs35713889: β =0.06, P =0.004 and rs3870341: β =0.03, P =0.001). LAMB2 encodes one of 15 subunits of Laminin, an extracellular matrix glycoprotein with a key role in the attachment, migration and organization of cells into tissues during embryonic development. Rare recessive mutations in LAMB2 cause Pierson’s syndrome (OMIM no. 609049), a disorder characterized by congenital nephrotic syndrome and ocular anomalies, typically with microcoria [5] ; neurological abnormalities are also described likely because of cortical laminar disorganization [6] . Common variants in/near other Laminin genes have been reported for a broad range of complex traits, including type 2 diabetes [7] , refractive error [8] , colorectal cancer [9] , IgG glycosylation [10] , ulcerative colitis [11] and coffee consumption [12] . A low-frequency missense variant in the TNRC6A gene was associated with later age at menarche (rs113388806; p.Q1112H; MAF 4.7%; β =0.08 years per allele; P =1.1 × 10 −11 ; Supplementary Fig. 3 ). This signal was only moderately well tagged by common HapMap2 SNPs (best proxy: rs12447003, r 2 =0.36, reported association with age at menarche: P =0.0005 (ref. 1 )). TNRC6A encodes an Argonaute-navigator protein, responsible for post-transcriptional gene silencing through RNA interference and microRNA pathways [13] . This finding further extends the range of epigenetic mechanisms implicated in the regulation of puberty [14] . A low-frequency missense variant in PRKAG1 was associated with earlier age at menarche (rs1126930; p.T98S; MAF 3.4%; β =−0.09 years per allele, P =9.6 × 10 −11 ; Supplementary Fig. 3 ). This low-frequency variant is only moderately well tagged by common HapMap2 SNPs (max r 2 =0.36), which reportedly showed subgenome-wide significant association with age at menarche (rs11837234, P =3.1 × 10 −6 ) [1] . This PRKAG1 missense variant is in the same locus as, but not correlated to, a reported [1] common signal for age at menarche (rs7138803, 848 kb apart, r 2 =0.02). PRKAG1 encodes the gamma-1 regulatory subunit of AMP-activated protein kinase, which senses and maintains cellular energy homeostasis by promoting fatty-acid oxidation and inhibiting fatty-acid synthesis; PRKAG1 is overexpressed in ovarian carcinomas [15] and is somatically mutated in colorectal cancers [16] . Our second genotyping approach considered X-chromosome GWAS SNPs in up to 76,831 women of European ancestry from the 23andMe study [17] . Imputation was performed against the 1000 Genomes reference, yielding genotype data for ∼ 266,000 X-chromosome variants (MAF>1%). Two signals, in/near IGSF1 and FAAH2 , reached genome-wide significance for association with age at menarche and both associations were confirmed in 39,486 independent women of European ancestry from the deCODE study. Common variants in and near IGSF1 were robustly associated with age at menarche (lead SNP: rs762080, MAF=24%; β =0.06 years per allele, P =9.4 × 10 −13 ; Supplementary Fig. 4 ). IGSF1 encodes the immunoglobulin superfamily member 1, which is a plasma membrane glycoprotein highly expressed in the pituitary gland and testis. Rare X-linked mutations in IGSF1 were recently described to cause central hypothyroidism, hypoprolactinemia, delayed puberty and macro-orchidism in males (OMIM no. 300888) [18] , [19] . Heterozygous female carriers reportedly had normal age at menarche; however, 6/18 had central hypothyroidism and 4/18 underwent oophorectomy for ovarian cysts [19] . The second X-chromosome locus, in Xp11.21 (lead SNP rs5914101 is intronic in FAAH2 , MAF 24%, β =0.05 years per allele, P =1.9 × 10 −10 ; Supplementary Fig. 4 ), lies within the critical region for Turner’s syndrome, which is the most common cause of primary ovarian insufficiency [20] . FAAH2 encodes fatty-acid amide hydrolase 2. This enzyme catalyses the hydrolysis and degradation of bioactive fatty-acid amides, a large class of endogenous signalling lipids including the endocannabinoids, which modulate several physiological processes, including feeding, inflammation, pain, sleep and various reproductive processes, including hypothalamic gonadotropin-releasing hormone secretion [21] , [22] . We sought to further functionally characterize the seven genes implicated by these analyses using expression data on 53 tissue types from the Genotype-Tissue Expression consortium [23] . All seven genes showed high relative tissue expression in the ovary and/or brain (specifically the hypothalamus; Supplementary Fig. 5 ); however, none of the lead SNPs showed a significant association with mRNA transcript abundance. None of the identified variants were associated with body mass index in 74,071 adults from the deCODE study (all P >0.05), indicating that their effects on puberty timing are unlikely to be mediated by body mass index. In summary, by large-scale analysis of genetic variation not captured by previous GWAS for age at menarche, we identified several low-frequency exonic variants of relatively large effect and two common X-chromosome signals. The implicated genes provide new insights into the mechanisms that link energy homeostasis to puberty timing, indicate possible roles of RNA-mediated gene silencing and fatty-acid amide signalling, and link genes behind rare autosomal, X-linked and syndromic disorders of puberty to normal variation in reproductive timing. Our findings using dense exome arrays in large unselected populations are informative for the clinical interpretation of heterozygous TACR3 variants in patients with rare disorders. In the deCODE study these novel variants collectively explained only 0.5% of the variance in age at menarche, suggesting that these often overlooked sources of genetic variation do not contribute disproportionately to the missing heritability of this complex trait. While variants with MAF below 1% are likely not well represented here, our findings indicate that, similar to other complex traits [24] , the genetic architecture of puberty timing is likely dominated by the additive effects of hundreds or even thousands of variants, each with relatively small effect. Exome array discovery analysis Exome array genotype data were generated across 19 studies in up to 76,657 women of genetically determined European ancestry with questionnaire-reported age at menarche between ages 9 and 17 years ( Supplementary Table 1 ). Exome array genotype calling for three studies (Framingham Heart Study (FHS), the Atherosclerosis Risk in Communities (ARIC) and Rotterdam Study (RS); totalling ∼ 9,000 women) was performed jointly as part of the CHARGE joint calling protocol [25] , which included over 62,000 individuals. Four additional studies (Cambridge Cancer, KORA, Korcula, Generation Scotland, total N ∼ 9,700) used the cluster file made available by CHARGE to call genotypes. Other studies followed standard calling and QC protocols for the Exome array ( Supplementary Table 2 ). Each contributing study ran a linear regression model on age at menarche, adjusted for birth year and principal components derived from genotypes, using the skatMeta/seqMeta package in R. Studies with family data included a random effect to account for relationships. Alleles were aligned to a common reference file before association testing (SNPInfo_HumanExome-12v1_rev5.tsv.txt available at http://www.chargeconsortium.com/main/exomechip/ ) and variants with MAF>5% in the meta-analysis were excluded. We performed gene-based testing (within seqMeta) for low-frequency variants using fixed effect burden tests, which assume that all rare variants have the same effect direction and size (scaled by a weight determined by allele frequency), and SKAT tests, which assume that rare variant effects are random and can contain a mixture of null, protective and risk rare alleles. These tests were run using three variant filters, all of which included only variants with MAF<1%: (1) all non-synonymous; (2) non-synonymous annotated as ‘damaging’ (conserved and predicted damaging, see http://www.chargeconsortium.com/main/exomechip/ ); and (3) only loss of function. The multiple testing adjustment included two tests × three filters × number of genes, requiring study-wise significance threshold P <1.14 × 10 −6 . For individual variants, a fixed-effects inverse variance-weighted meta-analysis was performed across all studies using METAL ( http://www.sph.umich.edu/csg/abecasis/Metal/ ), with associations considered significant at a conservative genome-wide significance threshold of P <5 × 10 −8 . Exome array follow-up studies We performed follow-up testing of selected exome array variants in the 23andMe study (as described below) and also in 39,486 independent women of European ancestry from the deCODE study, Iceland, who had genotypes on over 34 million variants by imputation of whole-genome sequencing-identified SNPs and indels on Illumina SNP chip data ( Supplementary Table 1 ) [26] . Variants from both studies were required to either pass genotyping QC (23andMe only, described below) or have imputation quality score >0.4. X-chromosome follow-up was performed in the deCODE study alone. All participants in all published studies provided informed consent, and the research protocol of each study was approved by their local research ethics committee [1] . 1000G X-chromosome discovery meta-analysis X-chromosome SNP data were generated in up to 76,831 women of European ancestry from the 23andMe study [17] , [27] , with questionnaire-reported age at menarche between the ages of 8 and 16 years, and who were genotyped on one or more of three GWAS arrays that also included customized content on human pathogenic variants ( Supplementary Table 1 ) [28] . 23andMe participants provided informed consent to take part in this research under a protocol approved by the AAHRPP-accredited institutional review board, Ethical and Independent Review Services. Before imputation, we excluded SNPs with Hardy–Weinberg equilibrium P <10 −20 , call rate <95% or with large allele frequency discrepancies compared with European 1000 Genomes reference data. Frequency discrepancies were identified by computing a 2 × 2 table of allele counts for European 1000 Genomes samples and 2,000 randomly sampled 23andMe customers with European ancestry, and identifying SNPs with a χ 2 P <10 −15 . Genotype data were imputed against the March 2012 ‘v3’ release of 1000 Genomes reference haplotypes. Age at menarche was assessed by questionnaire and recorded in 2-year-age bins, which were rescaled to 1-year effect estimates post analysis. The validity of this approach was confirmed by the lack of significant heterogeneity between rescaled 23andMe menarche estimates for the 123 previously identified signals and their reported effects [1] . Association results were obtained from linear regression models assuming additive allelic effects. These models included covariates for age and the top five GWAS SNP principal components to account for residual population structure. Results were further adjusted for a lambda genomic control value of 1.152 to correct for any residual test statistic inflation due to population stratification. Linkage disequilibrium score regression analysis (LDSC) [29] confirmed that principle component correction appropriately controlled for potential test statistic inflation due to population stratification (pre-genomic control-corrected calculated intercept ∼ 1). The reported association test P values were computed from likelihood ratio tests. X-chromosome follow-up Identified X-chromosome variants were replicated in 39,486 women from the deCODE study, as described above. How to cite this article: Lunetta, K. L. et al . Rare coding variants and X-linked loci associated with age at menarche. Nat. Commun . 6:7756 doi: 10.1038/ncomms8756 (2015).